Thetrans-SNARE-regulating function of Munc18-1 is essential to synaptic exocytosis The fusion of neurotransmitter-filled synaptic vesicles with the plasma membrane requires two classes of molecules—SNAP receptor (SNARE) and Sec1/Munc18 (SM) protein. Reconstitution studies suggest that the SM protein Munc18-1 promotes the zippering of trans -SNARE complexes and accelerates the kinetics of SNARE-dependent membrane fusion. However, the physiological role of this trans -SNARE-regulating function in synaptic exocytosis remains to be established. Here we first demonstrate that two mutations in the vesicle-anchored v-SNARE selectively impair the ability of Munc18-1 to promote trans -SNARE zippering, whereas other known Munc18-1/SNARE-binding modes are unaffected. In cultured neurons, these v-SNARE mutations strongly inhibit spontaneous as well as evoked neurotransmitter release, providing genetic evidence for the trans -SNARE-regulating function of Munc18-1 in synaptic exocytosis. Finally, we show that the trans -SNARE-regulating function of Munc18-1 is compromised by a mutation associated with Ohtahara Syndrome, a severe form of epilepsy. The release of neurotransmitters from chemical synapses is mediated by the fusion of membrane-bound synaptic vesicles with the plasma membrane. Intracellular vesicle fusion requires two conserved families of molecules—the soluble N -ethylmaleimide-sensitive factor attachment protein receptors (SNAP receptors or SNAREs), and the Sec1/Munc18 (SM) proteins [1] . The fusion reaction is initiated when the vesicle-rooted v-SNARE pairs with the target membrane-anchored t-SNAREs to form a trans -SNARE complex (also known as SNAREpin) [2] , [3] , [4] , [5] . The trans -SNARE complex zippers progressively towards the membrane-proximal domains [6] , [7] , forcing the two membrane bilayers into close apposition to fuse [8] , [9] . In synaptic vesicle fusion, syntaxin-1 and SNAP-25 serve as the t-SNAREs, whereas the cognate v-SNARE is VAMP2/synaptobrevin [2] , [10] , [11] , [12] , [13] . SM proteins are soluble factors of 60–70 kDa that control vesicle fusion through binding to their cognate SNAREs [14] , [15] , [16] , [17] . SM proteins display a similar knockout phenotype as that of SNAREs, and are essential for every vesicle fusion event in the cell [18] , [19] , [20] . In neurons, deletion of the synaptic SM protein Munc18-1 (also known as nSec1 or STXBP1) eliminates both spontaneous and evoked neurotransmitter release [21] , [22] , [23] , [24] . Although the mechanism of SNAREs is now well established, we are only beginning to understand how Munc18-1 regulates synaptic vesicle fusion. The first molecular target of Munc18-1 identified was the t-SNARE subunit syntaxin-1 (ref. 14 ). The syntaxin-1 monomer can adopt a ‘closed’ configuration when its N-terminal regulatory domain (Habc domain) folds back onto the C-terminal SNARE motif. Munc18-1 binds to the closed syntaxin-1 to form a heterodimer on the target membrane [25] , [26] , [27] , [28] . Although critical to the regulation of SNARE assembly [29] , [30] , this syntaxin-binding activity is not conserved among SM family proteins and is thought to represent an exocytosis-specific role of Munc18-1 (ref. 31 ). Thus, the regulation of synaptic release by Munc18-1 likely involves another mechanism that is independent of syntaxin monomer binding. Recently, it was discovered that Munc18-1 binds directly to the ternary SNARE complex assembled from the v-and t-SNAREs [32] , [33] . By recognizing the ternary SNARE complex, Munc18-1 promotes the zippering of trans -SNARE complexes and accelerates the kinetics of SNARE-dependent fusion reactions [32] , [34] , [35] . Munc18-1 selectively activates its cognate SNARE isoforms and therefore enhances vesicle fusion specificity [32] . The stimulatory function of Munc18-1 requires binding to the SNARE core bundle as well as the N-terminal peptide (N-peptide) motif, which is located at the extreme N terminus of syntaxin-1 (refs 32 , 33 , 34 , 35 ). Characterized by two or three charged residues followed by a hydrophobic leucine or phenylalanine residue, the N-peptide motif binds to a peripheral pocket on its cognate SM protein [36] , [37] . Although this trans -SNARE-regulating activity correlates well with Munc18-1’s essential role in synaptic release, the model is largely based on in vitro reconstitution experiments. Thus, the physiological relevance of the trans -SNARE-regulating function of Munc18-1 remains to be established. In this study, we designed genetic experiments to examine the trans -SNARE-regulating activity of Munc18-1 in synaptic exocytosis. Our strategy was to first make defined predictions regarding Munc18-1 function based on reconstitution experiments. We then tested the predictions in neurons using electrophysiological recordings. First, in a reconstituted system, we showed that two motifs on the v-SNARE VAMP2 are required for the stimulatory function of Munc18-1 in trans -SNARE zippering. Importantly, mutations of these VAMP2 motifs did not interfere with other known Munc18-1/SNARE-binding modes. In cultured neurons, the VAMP2 mutations strongly inhibited spontaneous as well as evoked neurotransmitter release. As a result, both excitatory and inhibitory synaptic transmissions were abolished. These genetic data strongly support that the trans -SNARE-regulating function of Munc18-1 has an essential role in synaptic exocytosis. Finally, we showed that a Munc18-1 mutation associated with Ohtahara Syndrome (OS), a severe form of epilepsy, compromises the ability of Munc18-1 to regulate the trans -SNARE complex in membrane fusion. Two VAMP2 mutations impair the trans -SNARE regulating function of Munc18-1 We previously showed that two motifs on VAMP2—S61/E62 and S75/Q76—are required for the stimulation of lipid mixing by Munc18-1 ( Fig. 1a ) [32] . These outward-facing motifs are conserved among synaptic exocytic v-SNAREs but are absent in non-cognate v-SNAREs such as the lysosomal v-SNARE VAMP8/endobrevin [32] . A true membrane fusion event is characterized by leakage-free merging of aqueous organelle contents (content mixing) [38] , [39] , [40] , whereas lipid mixing assays might monitor liposome juxtaposition rather than liposome fusion [41] . Thus, we first examined whether mutations of the two VAMP2 motifs impair the content mixing of the SNARE liposomes. 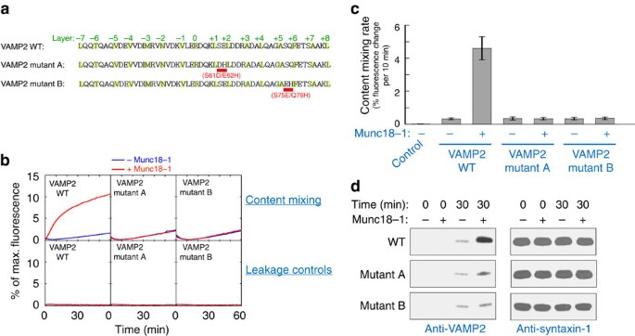Figure 1: Two VAMP2 mutations abrogate the stimulatory function of Munc18-1 in a reconstituted content-mixing reaction. (a) Sequences of the core domains of WT and mutant VAMP2 proteins. SNARE core layers are highlighted in green and numbered on the top. Two outward-facing motifs (marked by red bars) were substituted with their corresponding sequences in VAMP8, a non-cognate v-SNARE32. (b) Content mixing of the reconstituted fusion reactions. The soluble dye sulforhodamine B (50 mM) was encapsulated in the v-SNARE liposomes, in which its fluorescence was inhibited by self-quenching. The indicated v-SNARE liposomes were directed to fuse with unlabelled WT t-SNARE liposomes in the absence or presence of 5 μM Munc18-1. Each fusion reaction contained 5 μM t-SNAREs and 1.5 μM v-SNARE. In dequenching controls, the sulforhodamine B dye was included in both v- and t-SNARE liposomes. Data are presented as fluorescence increase over time. (c) Initial rates of the content-mixing reactions shown inb. In the control reaction, 20 μM of inhibitory VAMP2 CD was added to the fusion reaction reconstituted with WT SNAREs. Data are presented as percentage of fluorescence change per 10 min. Error bars indicate s.d. (d) Reconstituted t- and v-SNARE liposomes were incubated at 4 °C for the indicated periods in the presence or absence of 5 μM Munc18-1 before tenfold excess amount of VAMP2 CD was added to block unpaired t-SNAREs. The liposomes were subsequently solubilized and the t-SNAREs were precipitated using nickel beads. Presence of full-length VAMP2 in the precipitates was probed by immunoblotting, which was used as an indicator fortrans-SNARE assembly between liposomes. Figure 1: Two VAMP2 mutations abrogate the stimulatory function of Munc18-1 in a reconstituted content-mixing reaction. ( a ) Sequences of the core domains of WT and mutant VAMP2 proteins. SNARE core layers are highlighted in green and numbered on the top. Two outward-facing motifs (marked by red bars) were substituted with their corresponding sequences in VAMP8, a non-cognate v-SNARE [32] . ( b ) Content mixing of the reconstituted fusion reactions. The soluble dye sulforhodamine B (50 mM) was encapsulated in the v-SNARE liposomes, in which its fluorescence was inhibited by self-quenching. The indicated v-SNARE liposomes were directed to fuse with unlabelled WT t-SNARE liposomes in the absence or presence of 5 μM Munc18-1. Each fusion reaction contained 5 μM t-SNAREs and 1.5 μM v-SNARE. In dequenching controls, the sulforhodamine B dye was included in both v- and t-SNARE liposomes. Data are presented as fluorescence increase over time. ( c ) Initial rates of the content-mixing reactions shown in b . In the control reaction, 20 μM of inhibitory VAMP2 CD was added to the fusion reaction reconstituted with WT SNAREs. Data are presented as percentage of fluorescence change per 10 min. Error bars indicate s.d. ( d ) Reconstituted t- and v-SNARE liposomes were incubated at 4 °C for the indicated periods in the presence or absence of 5 μM Munc18-1 before tenfold excess amount of VAMP2 CD was added to block unpaired t-SNAREs. The liposomes were subsequently solubilized and the t-SNAREs were precipitated using nickel beads. Presence of full-length VAMP2 in the precipitates was probed by immunoblotting, which was used as an indicator for trans -SNARE assembly between liposomes. Full size image The soluble dye sulforhodamine B was encapsulated in the VAMP2 liposomes in which its fluorescence was inhibited by self-quenching [42] . Merging of the labelled VAMP2 liposomes with unlabelled t-SNARE liposomes led to the dilution and dequenching of sulforhodamine B fluorescence. We observed that the synaptic SNAREs drove a slow basal level of content mixing, which was strongly accelerated by Munc18-1 ( Fig. 1b,c ). The stimulatory activity of Munc18-1 in the content-mixing reaction was abrogated when either of the VAMP2 motifs was substituted with the corresponding sequences in the non-cognate v-SNARE VAMP8 (S61D/E62H and S75E/Q76H; Fig. 1b,c ). By contrast, the basal SNARE-mediated content mixing was not impacted by the VAMP2 mutations ( Fig. 1b,c ), suggesting that the pairing of the v- and t-SNAREs remained intact. To measure potential liposome leakage, the sulforhodamine B dye was loaded into both the v- and t-SNARE liposomes. In the absence of content leakage, no sulforhodamine B dequenching would be observed during the fusion reaction [42] . Indeed, the sulforhodamine B emission was not increased in these dequenching control reactions, indicating that there was no content leakage ( Fig. 1b ). Thus, true membrane fusion occurred in the reconstituted liposome fusion reactions. It was observed that, under certain experimental conditions, squid Munc18-1 could undergo denaturation and cause liposome aggregation, but these defects were not observed in mammalian Munc18-1 proteins [43] . We also found that recombinant mammalian Munc18-1 proteins (used in this study) were highly soluble and exhibited no noticeable aggregation. These content-mixing data establish that the two VAMP2 motifs—S61/E62 and S75/Q76—are essential to the stimulatory function of Munc18-1 in reconstituted fusion reactions. Next we sought to further determine how the VAMP2 mutations abolish the stimulatory function of Munc18-1 in membrane fusion. We first examined the effects of the mutations on membrane docking using a liposome docking assay. We observed that Munc18-1 only mildly increased the docking of SNARE liposomes ( Supplementary Fig. 1 ), consistent with our previous findings that SM proteins mainly act at a post-docking step of the fusion reaction [32] , [42] . Neither of the VAMP2 mutations significantly impacted the docking of the SNARE liposomes ( Supplementary Fig. 1 ). Next we tested how the VAMP2 mutations influence trans -SNARE zippering. In a trans -SNARE formation assay, which monitors the late stage of SNARE assembly, Munc18-1 strongly accelerated the assembly of trans -SNARE complexes between lipid bilayers ( Fig. 1d ). The stimulatory activity of Munc18-1 in trans -SNARE zippering was abolished when either of the VAMP2 motifs was mutated ( Fig. 1d ). The VAMP2 mutations did not reduce the basal level of trans -SNARE assembly (in the absence of Munc18-1; Fig. 1d ), consistent with the results of the basal content-mixing reactions ( Fig. 1b,c ). No liposome fusion was observed during the incubation period of the trans -SNARE formation reactions ( Supplementary Fig. 2 ). These data suggest that the two VAMP2 mutations abrogate the stimulatory function of Munc18-1 by impairing its ability to regulate trans -SNARE zippering. The binding of Munc18-1 to cis -SNARE complexes is not impacted by the VAMP2 mutations In addition to the trans -SNARE-regulating function, Munc18-1 also exhibits other SNARE-binding modes including association with the syntaxin monomer, the binary t-SNARE complex and the fully zippered cis -SNARE complex [32] , [33] , [44] . By nature, the binding of Munc18-1 to upstream targets—the syntaxin-1 monomer and the binary t-SNARE complex—does not involve the v-SNARE and therefore is not influenced by v-SNARE mutations. Next, we sought to define how the VAMP2 mutations impact the binding of Munc18-1 to the cis -SNARE complex. We used isothermal titration calorimetry (ITC) to measure the binding affinity between Munc18-1 and the cis -SNARE complex ( Fig. 2a ). Munc18-1 bound to the soluble form of synaptic cis -SNARE complex with a K d of ∼ 1.7 μM ( Fig. 2b ). Unexpectedly, neither of the VAMP2 mutations reduced the binding affinity between Munc18-1 and the cis -SNARE complex ( Fig. 2b ), in contrast to the strong effects of the mutations on the stimulatory function of Munc18-1 in trans -SNARE zippering. Thus, the two VAMP2 mutations selectively impair the ability of Munc18-1 to regulate the assembling trans -SNARE complex. Once the SNAREs become fully zippered, their association with Munc18-1 is no longer dependent on the two VAMP2 motifs. These findings also demonstrate that the Munc18-1/ cis -SNARE association cannot recapitulate the trans -SNARE-regulating function of Munc18-1 in the dynamic fusion reaction. 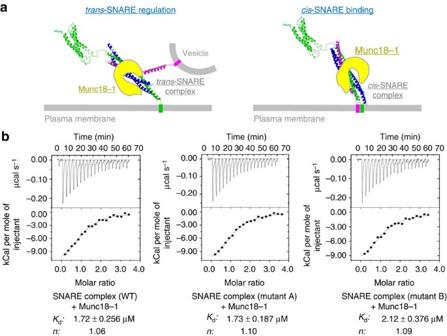Figure 2: The VAMP2 mutations do not interfere with the binding of Munc18-1 to the fully assembledcis-SNARE complex. (a) Schematic illustrations of thecis- andtrans-SNARE configurations. SNARE complexes were modelled from atomic structures35. (b) Ternary SNARE complexes were composed of t-SNARE CDs (syntaxin-1 (a.a. 1–265) and full-length SNAP-25) and VAMP2 CD (a.a. 1–95, WT or mutant). The VAMP2 mutants are illustrated inFig. 1a. Munc18-1 (5 μM) was loaded into the sample cell of the VP-ITC instrument, followed by the injection of SNARE complexes (75 μM) into the sample cell. The dissociation constant (Kd) and stoichiometry (n) of the interaction were calculated by fitting the data with a nonlinear least squares routine using the Microcal Origin software. Figure 2: The VAMP2 mutations do not interfere with the binding of Munc18-1 to the fully assembled cis -SNARE complex. ( a ) Schematic illustrations of the cis - and trans -SNARE configurations. SNARE complexes were modelled from atomic structures [35] . ( b ) Ternary SNARE complexes were composed of t-SNARE CDs (syntaxin-1 (a.a. 1–265) and full-length SNAP-25) and VAMP2 CD (a.a. 1–95, WT or mutant). The VAMP2 mutants are illustrated in Fig. 1a . Munc18-1 (5 μM) was loaded into the sample cell of the VP-ITC instrument, followed by the injection of SNARE complexes (75 μM) into the sample cell. The dissociation constant ( K d ) and stoichiometry ( n ) of the interaction were calculated by fitting the data with a nonlinear least squares routine using the Microcal Origin software. Full size image These results indicate that the two VAMP2 mutations did not impact any other known Munc18-1/SNARE-binding modes, and thus are uniquely suited for testing the physiological role of the trans -SNARE-regulating function of Munc18-1 in synaptic vesicle fusion. The VAMP2 mutants are correctly targeted to synaptic terminals To define how the VAMP2 mutations impact synaptic neurotransmitter release, lentivirus-based short hairpin RNAs (shRNAs) were introduced into cultured mouse neurons to silence VAMP2 expression ( Fig. 3a ). We tested multiple VAMP2 shRNAs and ultimately identified one highly effective shRNA that recognizes a 3′ untranslated region of the Vamp2 gene. Immunoblotting analysis showed that VAMP2 protein levels were reduced by >90% in the knockdown neurons ( Fig. 3b ). VAMP2 expression was restored by co-expression of shRNA-resistant Vamp2 rescue genes (wild-type (WT) or mutant). The WT and mutant VAMP2 proteins were expressed at comparable levels ( Fig. 3b ). 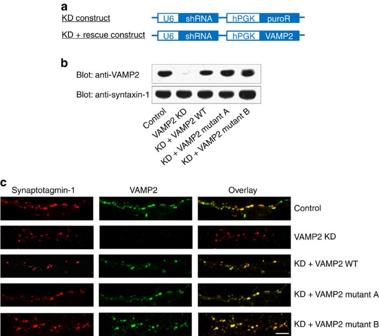Figure 3: The VAMP2 mutants are targeted correctly to synaptic terminals. (a) Diagrams showing the lentiviral shRNA constructs. In the knockdown (KD) construct, shRNA expression was driven by the U6 promoter, whereas the puroR gene was under the control of the hPGK promoter. In the KD and rescue construct, the puroR gene was replaced by the mouseVamp2gene. (b) Immunoblots showing the expression of VAMP2 and syntaxin-1 in the indicated neurons. Control: WT neurons with no lentiviral infection. (c) Representative immunostaining images showing the localization of WT and mutant VAMP2 proteins in synaptic terminals. Red: synaptotagmin-1; green: VAMP2. Scale bar, 5 μm. Figure 3: The VAMP2 mutants are targeted correctly to synaptic terminals. ( a ) Diagrams showing the lentiviral shRNA constructs. In the knockdown (KD) construct, shRNA expression was driven by the U6 promoter, whereas the puroR gene was under the control of the hPGK promoter. In the KD and rescue construct, the puroR gene was replaced by the mouse Vamp2 gene. ( b ) Immunoblots showing the expression of VAMP2 and syntaxin-1 in the indicated neurons. Control: WT neurons with no lentiviral infection. ( c ) Representative immunostaining images showing the localization of WT and mutant VAMP2 proteins in synaptic terminals. Red: synaptotagmin-1; green: VAMP2. Scale bar, 5 μm. Full size image Next, we examined the localization patterns of the VAMP2 proteins. We observed that both the WT and mutant VAMP2 proteins were concentrated at synaptic terminals, co-localizing with the synaptic vesicular protein synaptotagmin-1 ( Fig. 3c ). Therefore, the mutations did not interfere with the localization of the VAMP2 protein. Synaptotagmin-1 staining also indicates that the VAMP2 mutations do not alter synaptic densities in the cultured neurons ( Supplementary Fig. 3 ). The VAMP2 mutations inhibit neurotransmitter releases Next, we examined the effects of the VAMP2 mutations on spontaneous neurotransmitter release. Using electrophysiological recordings, we observed that VAMP2 knockdown severely diminished the frequency of spontaneous neurotransmitter release as monitored by the miniature excitatory postsynaptic currents (mEPSCs). WT VAMP2 fully rescued the knockdown phenotype, whereas the VAMP2 mutants did not ( Fig. 4a ). The amplitudes of mEPSCs were not altered by VAMP2 knockdown or mutations ( Fig. 4a ). Similarly, the frequency of miniature inhibitory postsynaptic currents (mIPSCs) was strongly reduced in VAMP2 knockdown neurons ( Fig. 4b ). The mIPSCs were restored by WT VAMP2 but not by the VAMP2 mutants. The amplitudes of mIPSCs remained unchanged ( Fig. 4b ). 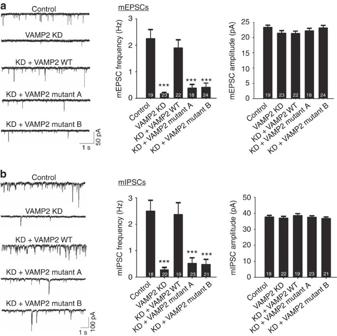Figure 4: The VAMP2 mutations strongly inhibit spontaneous neurotransmitter release. Cultured mouse cortical neurons were infected with lentiviruses expressing the VAMP2 shRNA (VAMP2 KD). In rescue experiments, neurons were infected with lentiviruses expressing both the VAMP2 shRNA and theVamp2rescue gene (KD+VAMP2 WT/mutant). The neurons are described inFig. 3. The VAMP2 mutants are illustrated inFig. 1a. (a) Spontaneous synaptic vesicle fusion monitored as miniature excitatory postsynaptic currents (mEPSCs). Left: representative traces of mEPSCs. Middle: summary graph of mEPSC frequency. Right: summary graph of mEPSC amplitudes. (b) Miniature inhibitory postsynaptic currents (mIPSCs). Left: representative traces of mIPSCs. Middle: summary graph of mIPSC frequency. Right: summary graph of mIPSC amplitudes. Data shown in summary graphs are means±s.em. Numbers of recorded cells are listed on the bars. Numbers of neurons and independent cultures are listed inSupplementary Table 1. Statistical analysis was performed using the Student’st-test comparing a test data set to the control experiment. ***P<0.001. Figure 4: The VAMP2 mutations strongly inhibit spontaneous neurotransmitter release. Cultured mouse cortical neurons were infected with lentiviruses expressing the VAMP2 shRNA (VAMP2 KD). In rescue experiments, neurons were infected with lentiviruses expressing both the VAMP2 shRNA and the Vamp2 rescue gene (KD+VAMP2 WT/mutant). The neurons are described in Fig. 3 . The VAMP2 mutants are illustrated in Fig. 1a . ( a ) Spontaneous synaptic vesicle fusion monitored as miniature excitatory postsynaptic currents (mEPSCs). Left: representative traces of mEPSCs. Middle: summary graph of mEPSC frequency. Right: summary graph of mEPSC amplitudes. ( b ) Miniature inhibitory postsynaptic currents (mIPSCs). Left: representative traces of mIPSCs. Middle: summary graph of mIPSC frequency. Right: summary graph of mIPSC amplitudes. Data shown in summary graphs are means±s.em. Numbers of recorded cells are listed on the bars. Numbers of neurons and independent cultures are listed in Supplementary Table 1 . Statistical analysis was performed using the Student’s t -test comparing a test data set to the control experiment. *** P <0.001. Full size image We then measured evoked neurotransmitter release in the cultured neurons. VAMP2 knockdown led to a strong reduction in the amplitudes of excitatory postsynaptic currents (EPSCs) triggered by local electrical stimulation. The defects in evoked responses were fully rescued by WT VAMP2 but not by the VAMP2 mutants ( Fig. 5a ). The amplitudes of the evoked inhibitory postsynaptic currents (IPSCs) were also dramatically reduced by VAMP2 knockdown. WT VAMP2 fully rescued IPSCs but the VAMP2 mutants did not ( Fig. 5b ). Thus, the two VAMP2 mutations abrogated evoked EPSCs and IPSCs. 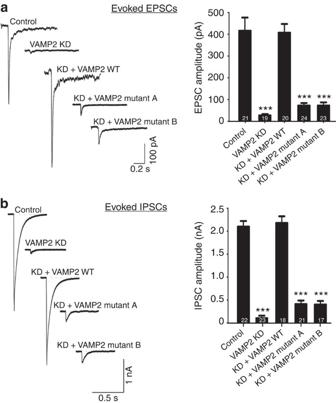Figure 5: Evoked neurotransmitter release is abolished by the VAMP2 mutations. (a) Left: representative traces of excitatory postsynaptic currents (EPSCs) evoked by local electrical stimulation in cultured neurons. Right: summary graph of EPSC amplitudes. (b) Left: representative traces of inhibitory postsynaptic currents (IPSCs) triggered by electrical stimulation. Right: summary graph of IPSC amplitudes. Data shown in the summary graphs are means±s.e.m. Numbers of recorded cells are listed on the bars. Numbers of neurons and independent cultures are listed inSupplementary Table 1. Statistical analysis was performed using the Student’st-test comparing a test data set to the control experiment. ***P<0.001. Figure 5: Evoked neurotransmitter release is abolished by the VAMP2 mutations. ( a ) Left: representative traces of excitatory postsynaptic currents (EPSCs) evoked by local electrical stimulation in cultured neurons. Right: summary graph of EPSC amplitudes. ( b ) Left: representative traces of inhibitory postsynaptic currents (IPSCs) triggered by electrical stimulation. Right: summary graph of IPSC amplitudes. Data shown in the summary graphs are means±s.e.m. Numbers of recorded cells are listed on the bars. Numbers of neurons and independent cultures are listed in Supplementary Table 1 . Statistical analysis was performed using the Student’s t -test comparing a test data set to the control experiment. *** P <0.001. Full size image We next examined the readily releasable pool (RRP) of synaptic vesicles. Applications of hypertonic sucrose solutions induced the exocytosis of synaptic vesicles resident in the RRP ( Supplementary Fig. 4 ). We observed that the RRP was strongly reduced in VAMP2 knockdown cells ( Supplementary Fig. 4 ). The RRP was restored by WT VAMP2 but not by the VAMP2 mutants ( Supplementary Fig. 4 ), indicating that the VAMP2 mutations impair the RRP of synaptic vesicles. To determine whether the VAMP2 mutations affect the Ca 2+ sensitivity of synaptic release, we recorded evoked responses at various extracellular Ca 2+ concentrations. We observed similar patterns of Ca 2+ responses in both WT and mutant neurons ( Supplementary Fig. 5 ), suggesting that the VAMP2 mutations do not impair the Ca 2+ -sensing machinery of synaptic release. Analysis using 10 Hz train stimulations suggests that the release probability of synaptic vesicles was reduced by the v-SNARE mutations ( Supplementary Fig. 6 ). RNA interference is often associated with off-target effects [45] . However, the fusion defects observed in the VAMP2 knockdown cells were similar to the phenotype of VAMP2 knockout neurons [46] , [47] . Moreover, neurotransmitter release was fully restored by the expression of the WT VAMP2 gene. Thus, we conclude that the VAMP2 shRNA inhibited synaptic neurotransmitter release by specifically ablating VAMP2 expression. Together, these results demonstrate that the VAMP2 mutations strongly inhibit both spontaneous and evoked neurotransmitter release in cultured neurons. As a result, both excitatory and inhibitory synaptic transmissions are abolished. These genetic data confirm the findings of the reconstitution experiments and provide direct evidence for the trans -SNARE-regulating function of Munc18-1 in synaptic vesicle fusion. An OS-causing mutation impairs the trans -SNARE-regulating function of Munc18-1 OS, also known as early infantile epileptic encephalopathy, is one of the severest forms of epilepsy characterized by early onset of intractable tonic spasms and developmental retardation [48] , [49] . De novo heterozygous STXBP1 (the human gene that encodes the Munc18-1 protein) mutations are frequently found in OS patients. Proteins encoded by the mutated STXBP1 allele are unable to regulate synaptic transmission. Molecules encoded by the WT STXBP1 allele are functional but their quantities are inadequate in maintaining full synaptic activities in humans ( STXBP1 haploinsufficiency). Importantly, STXBP1 haploinsufficiency impairs the inhibitory synaptic transmission more than the excitatory synaptic transmission, resulting in improper neuronal excitation observed in OS patients [49] , [50] , [51] , [52] , [53] . It remains unclear how Munc18-1 function is affected by OS-causing mutations. As STXBP1 haploinsufficiency causes OS, the question now becomes how STXBP1 mutations impair the function of Munc18-1 in synaptic release. Our reconstituted fusion system provides a platform in which the functional consequence of a Munc18-1 mutation can be causally established. Here, we focused on a single base pair mutation in the STXBP1 gene that results in the substitution of the cysteine 552 residue with an arginine (C552R) in the Munc18-1 protein ( Fig. 6a ) [53] . The cysteine 552 residue is located at the C-terminal Domain 2 of the Munc18-1 protein [25] , [54] . Circular dichroism measurements indicate that the overall folding of the C552R mutant was similar to that of the WT protein ( Fig. 6b ). In line with this notion, the C552R mutant bound to the syntaxin-1 monomer as well as WT Munc18-1 ( Fig. 6c ). Interestingly, local near ultraviolet scans revealed minor but clear differences between the WT and mutant proteins ( Supplementary Fig. 7 ), suggesting that the C552R mutation causes subtle domain rearrangements in Munc18-1. 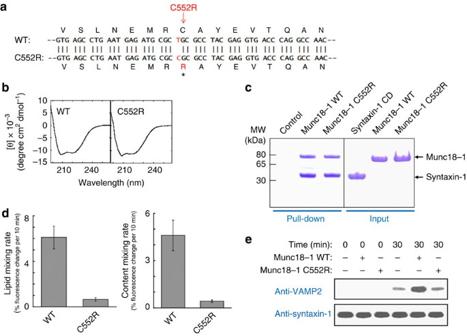Figure 6: A Munc18-1 mutation associated with the Ohtahara Syndrome interferes with itstrans-SNARE-regulating function. (a) Sequences showing the single base pair mutation in theSTXBP1gene that resulted in the substitution of the cysteine 552 residue with an arginine (C552R). (b) Circular dichroism (CD) spectroscopic analysis of WT and mutant Munc18-1 proteins. The CD spectra were measured using a Jasco J-815 spectropolarimeter equipped with a 1-mm quartz cell. The readings were made at 0.1 nm intervals, and each data point represented the average of six scans at a speed of 50 nm min−1over the wavelength range of 200–260 nm. (c) The binding of Munc18-1 to syntaxin-1 monomer. His6-SUMO-tagged Munc18-1 proteins (WT or C552R mutant) were immobilized on nickel agarose beads (Qiagen), and were used to pull down syntaxin-1 (a.a. 1–262). After incubation at 4 °C for 1 h, the beads were washed three times with the protein-binding buffer (see the ITC method). Subsequently, the bound protein complexes were resolved on SDS–PAGE and stained with coomassie blue. (d) Initial rates of the SNARE-Munc18-1-mediated lipid-mixing (left) and content-mixing (right) reactions. Each reaction contained 5 μM t-SNAREs, 1.5 μM v-SNARE and 5 μM Munc18-1 (WT or C552R mutant). Data are presented as percentage of fluorescence change per 10 min. Error bars indicate s.d. (e) The Munc18-1 C552R mutant was defective in promotingtrans-SNARE assembly. Figure 6: A Munc18-1 mutation associated with the Ohtahara Syndrome interferes with its trans -SNARE-regulating function. ( a ) Sequences showing the single base pair mutation in the STXBP1 gene that resulted in the substitution of the cysteine 552 residue with an arginine (C552R). ( b ) Circular dichroism (CD) spectroscopic analysis of WT and mutant Munc18-1 proteins. The CD spectra were measured using a Jasco J-815 spectropolarimeter equipped with a 1-mm quartz cell. The readings were made at 0.1 nm intervals, and each data point represented the average of six scans at a speed of 50 nm min −1 over the wavelength range of 200–260 nm. ( c ) The binding of Munc18-1 to syntaxin-1 monomer. His 6 -SUMO-tagged Munc18-1 proteins (WT or C552R mutant) were immobilized on nickel agarose beads (Qiagen), and were used to pull down syntaxin-1 (a.a. 1–262). After incubation at 4 °C for 1 h, the beads were washed three times with the protein-binding buffer (see the ITC method). Subsequently, the bound protein complexes were resolved on SDS–PAGE and stained with coomassie blue. ( d ) Initial rates of the SNARE-Munc18-1-mediated lipid-mixing (left) and content-mixing (right) reactions. Each reaction contained 5 μM t-SNAREs, 1.5 μM v-SNARE and 5 μM Munc18-1 (WT or C552R mutant). Data are presented as percentage of fluorescence change per 10 min. Error bars indicate s.d. ( e ) The Munc18-1 C552R mutant was defective in promoting trans -SNARE assembly. Full size image Next, we examined how the C552R mutation affects the stimulatory function of Munc18-1 in membrane fusion. When added to a reconstituted lipid-mixing assay, the Munc18-1 C552R mutant was defective in stimulating SNARE-mediated lipid mixing ( Fig. 6d ). Similarly, the C552R mutant was unable to accelerate the SNARE-mediated content mixing reaction ( Fig. 6d ). In a trans -SNARE formation assay, the Munc18-1 C552R mutant failed to accelerate trans -SNARE zippering ( Fig. 6e ). By contrast, the mutation did not reduce the binding of Munc18-1 to the cis -SNARE complex in solution ( Supplementary Fig. 8 ), consistent with the notion that cis -SNARE binding does not recapitulate the activity of Munc18-1 in the fusion reaction. These results demonstrate that the C552R mutation selectively compromises the trans -SNARE-regulating function of Munc18-1 in membrane fusion, providing a molecular explanation for the OS-causing mutation. In patients harbouring the heterozygous C552R mutation, only half of the expressed Munc18-1 proteins are active, which is expected to compromise synaptic balance due to STXBP1 haploinsufficiency. As STXBP1 haploinsufficiency impairs the inhibitory synaptic transmission more than the excitatory synaptic transmission, the mutation results in dysregulated neuronal excitation in the OS patients. Compositionally defined systems reconstituted with purified components are designed to reveal the intrinsic activities of molecules without the complications of other factors naturally present in the cell. In reconstituted assays, Munc18-1 promotes the zippering of trans -SNARE complexes and strongly accelerates the kinetics of SNARE-mediated membrane fusion [32] , [34] , [35] , [55] , [56] , [57] , [58] , [59] , [60] , [61] . This trans -SNARE-regulating function likely represents a conserved mechanism of SM family proteins [42] , [62] . A model derived from reconstituted assays, however, should be considered as a theory that must be tested in a physiological setting. A major gap in the studies of Munc18-1 is the dearth of direct genetic evidence for its trans -SNARE-regulating function in synaptic exocytosis. To determine the physiological role of this trans -SNARE-regulating function, it is imperative to distinguish it from other known Munc18-1/SNARE-binding modes. In this work, we succeeded in this goal by identifying two motifs in the v-SNARE VAMP2—S61/E62 and S75/Q76—that are only required for the trans -SNARE-regulating function of Munc18-1 in membrane fusion. Our electrophysiological measurements demonstrated that mutations of the VAMP2 motifs strongly inhibit spontaneous as well as evoked neurotransmitter release in cultured neurons, thus confirming the findings of the reconstitution experiments. The regulation of trans -SNARE complexes by Munc18-1 is a highly dynamic process. Therefore, we cannot directly assess whether the two VAMP2 mutations physically interact with Munc18-1 in the context of the trans -SNARE complex. It remains possible that the VAMP2 mutations interfere with Munc18-1 activities indirectly by altering the spatial configuration of the trans -SNARE complex such that it is no longer compatible with Munc18-1 function. In addition, we cannot completely rule out the possibility that the VAMP2 mutations also impair a Munc18-1-independent function in neurons. However, two independent VAMP2 motifs were tested in this study and it is highly unlikely that the two VAMP2 motifs could be both engaged in the regulatory activity of another synaptic molecule. Moreover, the consequences of the VAMP2 mutations in synaptic vesicle fusion match well with their effects on Munc18-1 function in vitro . Thus, we conclude that the VAMP2 mutations abrogate neurotransmitter release by selectively impairing the ability of Munc18-1 to regulate the trans -SNARE complex. Further evidence for the trans -SNARE-regulating function of Munc18-1 is provided by our analysis of a heterozygous Munc18-1 mutation associated with OS. Because of STXBP1 haploinsufficiency [48] , loss-of-function mutations in one allele of the STXBP1 gene cause imbalances in synaptic networks. Certain OS-associated Munc18-1 mutations appear to result in the collapse of Munc18-1 structure [48] , [52] . By contrast, the overall architecture of the C552R mutant remains intact but the mutation compromises the ability of Munc18-1 to regulate trans -SNARE complexes. As STXBP1 haploinsufficiency impairs the inhibitory synaptic transmission more than the excitatory synaptic transmission, these loss-of-function mutations are expected to cause improper neuronal excitation, a hallmark of OS. As more OS-associated Munc18-1 mutations are identified, we anticipate that defects in trans -SNARE regulation likely represent a common mechanism for OS pathogenesis. SNAREs and SM proteins are conserved molecules that mediate all vesicle fusion pathways in the cell. In synaptic vesicle fusion, SNAREs and Munc18-1 are superimposed by specialized factors, including synaptotagmin, complexin, Munc13 and CAPS, to allow for temporal and spatial regulation [29] , [63] , [64] , [65] , [66] , [67] , [68] . Our data showed that both spontaneous and evoked synaptic releases are abolished when the trans -SNARE-regulating function of Munc18-1 is impaired. Therefore, although we did not directly investigate the exocytosis-specific factors, the mechanism of Munc18-1 revealed in minimal systems is also valid in the presence of these molecules in neurons. Recombinant protein expression and purification Recombinant t-and v-SNARE proteins were expressed in Escherichia coli and purified by nickel affinity chromatography. The synaptic t-SNARE complex was composed of His 6 -SNAP-25 and untagged syntaxin-1. The v-SNARE VAMP2 possessed no extra residues after the tag was proteolytically removed [34] . SNAREs were stored in a buffer containing 25 mM HEPES (pH 7.4), 400 mM KCl, 1% n -octyl-β- D -glucoside (Calbiochem), 10% glycerol (v/v) and 0.5 mM Tris(2-carboxyethyl)phosphine (Gold Biotechnology). The cytoplasmic domains (CDs) of SNAREs were purified using the same procedures as the WT proteins except that detergents were not included. Recombinant Munc18-1 proteins were expressed and purified from E. coli . The bacteria were grown at 37 °C until the optical density reached 0.6. Subsequently the temperature was lowered to 16 °C and 0.2 mM isopropyl-β- D -thiogalactoside was added to induce Munc18-1 expression. After 16 h, the bacteria were harvested and Munc18-1 proteins were purified using affinity chromatography. SNARE and Munc18-1 mutants were generated by site-directed mutagenesis (Stratagene/Agilent Technologies), and purified similarly to the corresponding WT proteins. Reconstitution of proteoliposomes All lipids were acquired from Avanti Polar Lipids Inc. To prepare v- and t-SNARE liposomes, 1-palmitoyl-2-oleoyl-sn-glycero-3-phosphocholine, 1-palmitoyl-2-oleoyl-sn-glycero-3-phosphoethanolamine, 1-palmitoyl-2-oleoyl-sn-glycero-3-phosphoserine and cholesterol were mixed in a molar ratio of 60:20:10:10. SNARE proteoliposomes were prepared by detergent dilution [69] , [70] . To prepare liposomes for content-mixing assays, v-SNARE liposomes were reconstituted in the presence of 50 mM sulforhodamine B (Sigma). Detergents and free sulforhodamine B were removed from the samples by overnight dialysis using dialysis tubes (Novagen) against the reconstitution buffer (25 mM HEPES (pH 7.4), 100 mM KCl, 10% glycerol (v/v) and 1 mM dithiothreitol), followed by flotation on a Nycodenz (Axis-Shield) density gradient. The molar protein/lipid ratio was 1:200 for v-SNAREs, and 1:500 for t-SNARE liposomes. Only freshly prepared liposomes were used in content mixing reactions. The size and purity of the reconstituted proteoliposomes were monitored by dynamic light scattering and analytical nycodenz gradient flotation ( Supplementary Fig. 9 ). Liposome fusion assays Content-mixing reactions contained 45 μl of unlabelled t-SNARE liposomes and 5 μl of sulforhodamine B-loaded v-SNARE liposomes in which the sulforhodamine B fluorescence was inhibited by self-quenching. The fusion reactions were carried out at 37 °C in the reaction buffer (25 mM HEPES (pH 7.4), 100 mM KCl and 1 mM dithiothreitol) in a 96-well plate (Nunc). Merging of the liposomes resulted in the mixing of their contents and the dequenching of sulforhodamine B. The increase of sulforhodamine B fluorescence at 585 nm (excitation 565 nm) was measured every two minutes in a BioTek Synergy HT microplate reader. At the end of the reaction, 10 μl of 2.5% dodecyl-maltoside (w/v, Roche) was added to the liposomes [35] , [42] . To assess Munc18-1 activity, SNARE liposomes were preincubated with Munc18-1 or protein buffer for 1 h at 4 °C. Content-mixing data are presented as the percentage of maximum fluorescence change. The maximum rate within the first 10 min of the reaction was used to represent the initial rate of a liposome fusion reaction. In reactions with decreases in initial fluorescence (because of temperature change), the phase of fluorescence decrease was omitted from the calculations. Full accounting of statistical significance was included for each data set based on at least three independent experiments. Trans -SNARE formation assay Reconstituted t- and v-SNARE liposomes were incubated at 4 °C in the presence or absence of 5 μM Munc18-1 before ten-fold excess amount of inhibitory VAMP2 CD was added. The liposomes were solubilized with 1% CHAPS, and the t-SNAREs were precipitated using nickel beads (through binding to His 6 -SNAP-25). Presence of full-length VAMP2 in the precipitates was probed by immunoblotting using monoclonal anti-VAMP2 antibodies (1:2,000 dilution; Synaptic Systems, Cat#104 211), which was used as an indicator for trans -SNARE formation between liposomes. Syntaxin-1 was detected using monoclonal anti-syntaxin-1 antibodies (1:1,000 dilution; Synaptic Systems, Abcam, Cat#ab3265). ITC measurements ITC measurements were performed at 25 °C using a VP-ITC instrument (Microcal). All recombinant proteins were dialysed overnight in a binding buffer (25 mM HEPES (pH 7.4), 150 mM KCl, 10% glycerol (v/v) and 0.5 mM Tris(2-carboxyethyl)phosphine). SNARE complexes were prepared by incubating t-SNARE CDs (syntaxin-1 (amino acids (a.a.) 1–265) and full-length SNAP-25) with VAMP2 CD (a.a. 1–95) and Vc peptide (a.a. 57–92) overnight at 4 °C in the binding buffer. The assembled SNARE complexes were purified by gel filtration chromatography. Munc18-1 (5 μM) was loaded into the sample cell of the VP-ITC instrument, followed by the injection of SNARE complexes (75 μM) into the sample cell. After polynomial baseline corrections to remove the slight drifts in initial data points, the data were fitted with a nonlinear least squares routine using the Microcal Origin software. Primary neuron culture and lentiviral infection Cortical neurons were isolated from newborn C57BL/6 mice (Jackson Laboratory). The cells were dissociated by papain (Worthington) digestion and plated on glass coverslips coated with poly- D -lysine (Sigma). The neurons were maintained in the Neurobasal medium (Life Technologies) supplemented with B-27 (Life Technologies), glutaMAX (Life Technologies) and Ara-C (Sigma) according to the Life Technologies’ instructions. All mice were handled according to the NIH guidelines for Animal Care and Use, and the procedures were approved by the Institutional Animal Care and Use Committee at the University of Colorado-Boulder. To silence VAMP2 expression in neurons, a Vamp2 -targeting lentiviral shRNA plasmid (TRCN0000110540, Sigma) was obtained from the University of Colorado Functional Genomics Facility. The shRNA targets a 21-bp sequence (5′-CCGACCACAATCTGGTTCTTT-3′) in the 3′ untranslated region of the mouse Vamp2 gene. To introduce the rescue Vamp2 gene, the lentiviral shRNA plasmid was digested with Bam HI and Kpn I to remove the puromycin resistance gene (puroR). Mouse Vamp2 gene was subcloned into the Bam HI and Kpn I sites of the lentiviral vector such that its expression was driven by the hPGK promoter. These constructs allowed for simultaneous expression of the Vamp2 shRNA and the Vamp2 rescue gene. VAMP2 mutations were introduced by site-directed mutagenesis. Knockdown efficiency and rescue gene expression were examined by immunoblotting. To produce lentiviral particles, lentiviral expression plasmids were transfected into HEK 293 T cells along with helper plasmids—pCMV-VSVG, psPAX2 and pAdVAntage. Forty-eight hours after transfection, cell culture supernatants containing lentiviral particles were collected and filtered through 0.45 μm syringe filters (Corning). The supernatants were concentrated by centrifugation at 25,000 r.p.m. for 1 h in a Beckman SW28 rotor (Beckman). Neurons were infected with the lentiviruses at DIV 6, and analysed by electrophysiological measurements at DIV 16–20. Immunoblotting and immunostaining For immunoblotting, cellular proteins were extracted by SDS sample buffer and resolved on SDS–PAGE. After being transferred onto PVDF membranes, VAMP2 and syntaxin-1 were probed as described in the trans -SNARE formation assay. Protein levels were quantified using the ImageJ software (National Institutes of Health). Original immunoblots are included in Supplementary Fig. 10 . For immunostaining, cells were fixed by 4% paraformaldehyde (Sigma) and permeabilized using 0.2% Triton X-100. After blocking with 10% BSA, VAMP2 was detected by monoclonal anti-VAMP2 antibodies (1:500 dilution) and goat Fluor 488-conjugated secondary antibodies (1:200 dilution; Life Technologies, Cat#A-11001). Synaptotagmin-1 was detected by rabbit polyclonal anti-synaptotagmin-1 antibodies (1:1,000 dilution; a gift from James Rothman lab) and goat rhodamine-conjugated secondary antibodies (1:200 dilution; Jackson ImmunoResearch, Cat#111-025-003). Images were acquired on a Carl Zeiss 3i Marianas spinning disk confocal microscope unless otherwise stated, and processed using ImageJ. Electrophysiological recordings Evoked synaptic transmission was triggered by one millisecond current injections using a concentric bipolar microelectrode (FHC; Model: CBAEC75) placed about 100–150 μm from the cell bodies of patched neurons. The extracellular stimuli were manipulated using an Isolated Pulse Stimulator (World Precision Instruments). The evoked responses were measured by whole-cell recordings using a Multiclamp 700B amplifier (Molecular Devices). The whole-cell pipette solution contained 135 mM CsCl, 10 mM HEPES-CsOH (pH 7.25), 0.5 mM EGTA, 2 mM MgCl 2 , 0.4 mM NaCl-GTP and 4 mM NaCl-ATP. The bath solution contained 140 mM NaCl, 5 mM KCl, 2 mM CaCl 2 , 0.8 MgCl 2 , 10 mM HEPES-NaOH (pH 7.4) and 10 mM glucose. EPSCs and IPSCs were distinguished by including 50 μM picrotoxin or 20 μM 6-cyano-7-nitroquinoxaline-2,3-dione (CNQX) and 50 μM DL-2-amino-5-phosphonopentanoic acid (AP-5) (all from Sigma), respectively, in the bath solution. The mEPSCs and mIPSCs of the neurons were sampled at 10 kHz in the presence of 1 μM tetrodotoxin (Sigma). The resistance of pipettes was 3-5 mega ohms. The series resistance was adjusted to 8–10 mega ohms once the whole-cell configuration was established. Sucrose-evoked synaptic release was triggered by a 5-s application of 0.5 M sucrose in the presence of AP-5, CNQX and tetrodotoxin, puffed by Picospritzer III (Parker). The detailed numbers of cultures and neurons are listed in Supplementary Table 1 . The electrophysiological data were analysed using the pClamp 10 software (Molecular Devices). For statistical calculations, all data are shown as means±s.e.m. The P values were calculated using Student’s t -test. In gene rescue experiments, all data are compared with control WT neurons. How to cite this article: Shen, C. et al . The trans -SNARE-regulating function of Munc18-1 is essential to synaptic exocytosis. Nat. Commun. 6:8852 doi: 10.1038/ncomms9852 (2015).